Human haemodynamic frequency harmonics regulate the inflammatory phenotype of vascular endothelial cells Haemodynamic variations are inherent to blood vessel geometries (such as bifurcations) and correlate with regional development of inflammation and atherosclerosis. However, the complex frequency spectrum characteristics from these haemodynamics have never been exploited to test whether frequency variations are critical determinants of endothelial inflammatory phenotype. Here we utilize an experimental Fourier transform analysis to systematically manipulate individual frequency harmonics from human carotid shear stress waveforms applied in vitro to human endothelial cells. The frequency spectrum, specifically the 0th and 1st harmonics, is a significant regulator of inflammation, including NF-κB activity and downstream inflammatory phenotype. Further, a harmonic-based regression-model predicts eccentric NF-κB activity observed in the human internal carotid artery. Finally, short interfering RNA-knockdown of the mechanosensor PECAM-1 reverses frequency-dependent regulation of NF-κB activity. Thus, PECAM-1 may have a critical role in the endothelium’s exquisite sensitivity to complex shear stress frequency harmonics and provide a mechanism for the focal development of vascular inflammation. It has long been appreciated that shear stresses generated by complex haemodynamic blood flow impact blood vessel health and function. These shear stresses naturally vary due to changes in vessel wall geometry, creating region-specific phenotypic differences in the endothelial cells (ECs) lining the vessel walls. This drives the localization, formation and progression of the inflammatory disease, atherosclerosis [1] , [2] . For instance, these focal inflammatory responses are typically found in areas of bifurcations or bulbous regions that have low shear stress magnitudes and often flow reversals—in these unique regions, blood flow forces ‘prime’ the endothelium towards inflammation and atherosclerosis (atheroprone). A hallmark of this response is increased activity of the inflammatory transcription factor, nuclear factor-κB (NF-κB) and expression of adhesion molecules. Conversely, shear stresses within straight regions of the vasculature are generally higher, unidirectional and promote mechanisms that thwart inflammation (atheroprotective), such as KLF2 and KLF4 expression [3] , [4] , [5] , [6] , [7] . Further, lesions often develop eccentrically along the vessel wall mere centimeters away from regions that do not develop disease—this suggests that ECs are exquisitely sensitive to small regional changes in haemodynamics that have large impacts on vessel wall inflammation. Owing to the complex nature of time-varying (pulsatile) blood flow patterns, it is difficult to decouple the haemodynamic characteristics that drive cellular phenotype and disease development. Such differences may include shear stress magnitude, direction, temporal gradients and frequency content [8] , [9] , [10] , [11] . One important observation is that ECs exposed to steady flows (lacking frequency content) differ from those exposed to pulsatile flows (containing frequency content), suggesting that frequency content may be an important regulator of EC phenotype [12] . Indeed, some evidence shows that sinusoidal shear stresses of different frequencies regulate endothelial nitric oxide synthase (eNOS), cell proliferation and many inflammatory genes [8] , [13] , [14] . Himburg et al. [8] reported that bovine EC expression of many inflammatory genes was differentially activated between 1, 2 or 3 Hz of sinusoidal flow. An important limitation, however, is that, like many biophysical stimuli, in vivo human shear stress waveforms are more complex—simultaneously composed of numerous frequency harmonics with amplitudes that vary in several orders of magnitude [15] . Our lab and others found that physiological shear stresses (composed of a full spectrum of in vivo harmonics) influence EC migration, ER stress, matrix deposition, permeability and inflammatory signalling that translate to in vivo biology [5] , [16] , [17] , [18] , [19] , [20] , [21] , [22] , [23] , [24] . Many of these responses are dependent on platelet endothelial cell adhesion molecule-1 (PECAM-1) that forms a mechanosensory complex [25] . In ApoE−/− mice, we showed that PECAM-1 contributes to atherosclerosis development in disease-prone regions, where it was necessary for the sustained, region-specific activation of NF-κB and fibronectin (FN) deposition [22] , [23] , [24] , [26] , [27] , [28] . Shear stress characteristics previously found to impact EC biology in isolation (time-averaged magnitude, direction, temporal gradients and frequency content) can be fundamentally described by the frequency spectrum. Herein we merge common mathematical tools from the field of electrical engineering with biology to systematically test the role of frequency harmonics from complex shear stress patterns on EC phenotype. We hypothesize that shear stress frequency components regulate the endothelial inflammatory phenotype, and that PECAM-1 is a critical mediator of this response. Haemodynamics in vitro translates to in vivo biology In the carotid bifurcation, inflammation and atherosclerosis typically occur within internal carotid sinus (ICS) where blood flow velocity ( U z ) and wall shear stress ( τ w ) are lower compared with the common carotid artery (CCA). Additionally, this region has an elevated oscillatory shear index (OSI) and harmonic index (HI), which correlate with atherosclerosis [15] , [29] . 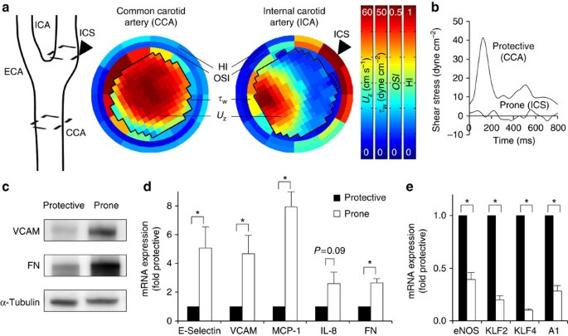Figure 1: Carotid artery atheroprone and atheroprotective shear stress waveforms evoke distinct endothelial phenotypes. (a) Previously blood flow velocities (Uz) from the internal and common carotid arteries were measured. Using this information, the haemodynamic parameters wall shear stress (τw), oscillatory shear index (OSI) and the harmonic index (HI) were computed between these different regions circumferentially around the blood vessel. (b) Atheroprone and atheroprotective shear stress waveforms from the human internal carotid sinus (ICS) and common carotid artery (CCA), respectively, were appliedin vitroto confluent ECs for 24 h. Pro-inflammatory proteins (c) and gene expression (d) were elevated under atheroprone flow, while the opposite was seen with anti-inflammatory genes (e). Statistics: *P<0.05 for Student’s one-samplet-test,N=4–10. Figure 1a illustrates the regional and circumferential differences in atheroprone haemodynamics (ICS) compared with the atheroprotective, CCA, by showing the velocity within the lumen at peak systole, along with differences in haemodynamics parameters around the vessel wall. Our haemodynamic device can accurately apply these in vivo waveforms in vitro ( Fig. 1b ) to ECs, where after 24 h, the cells reprogramme to acquire distinct phenotypes that are representative of the regional in vivo biology ( Fig. 1c–e ) [5] , [16] , [17] , [23] . Atherogenic, NF-κB-dependent proteins, vascular adhesion molecule (VCAM) and FN, were increased under atheroprone (prone) shear stress compared with atheroprotective (protective) ( Fig. 1c ). Similar to previous studies, we found that NF-κB activity and downstream gene expression (E-Selectin, VCAM, MCP-1 (monocyte chemoattractant protein-1), IL-8 (interleukin-8), FN) was increased under prone compared with protective haemodynamics ( Fig. 1d ) [4] , [30] , [31] . Conversely, known antiatherogenic/prosurvival genes (eNOS, KLF2, KLF4 and BCL2-like protein A1 (A1)) were upregulated in response to protective haemodynamics [3] , [5] , [32] , [33] , [34] ( Fig. 1e ). These responses are consistent with those from human aortic ECs ( Supplementary Fig. S1 ), and more importantly, mirror those found in the human carotid arteries, from which the haemodynamic waveforms were derived. Figure 1: Carotid artery atheroprone and atheroprotective shear stress waveforms evoke distinct endothelial phenotypes. ( a ) Previously blood flow velocities ( U z ) from the internal and common carotid arteries were measured. Using this information, the haemodynamic parameters wall shear stress ( τ w ), oscillatory shear index (OSI) and the harmonic index (HI) were computed between these different regions circumferentially around the blood vessel. ( b ) Atheroprone and atheroprotective shear stress waveforms from the human internal carotid sinus (ICS) and common carotid artery (CCA), respectively, were applied in vitro to confluent ECs for 24 h. Pro-inflammatory proteins ( c ) and gene expression ( d ) were elevated under atheroprone flow, while the opposite was seen with anti-inflammatory genes ( e ). Statistics: * P <0.05 for Student’s one-sample t -test, N =4–10. Full size image The frequency spectrum regulates inflammatory pathways It is unclear what the dominant haemodynamic characteristics are that determine in vivo vascular phenotype. To address this problem, we applied a common practice from signal processing—the Fourier Transform (FT). All signals can be represented as a summation of sinusoid waveforms of differing amplitude and frequency. Performing a FT on a periodic signal yields an equivalent signal represented as a discrete frequency spectrum that gives the amplitudes of individual harmonics (multiples of the fundamental frequency which is the heart-rate of 1.25 Hz). 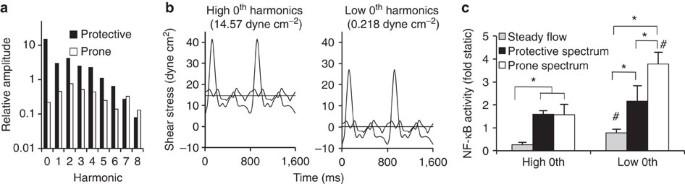Figure 2: Atheroprone and atheroprotective frequency spectrums regulate NF-κB activity. (a) Fourier transform analysis was performed on the protective and prone waveforms. (b) The corresponding 0th harmonic (time-average shear stress) from the prone (low 0th) and protective (high 0th) was held constant, while exchanging the higher frequency spectrum from the prone or protective waveforms, or compared with steady flow lacking harmonic content. (c) After 24 h of shear stress, NF-κB activity was assessed. Statistics: *P<0.05 for one-way ANOVA,N=8–10,#P<0.05 for Student’st-test compared with equivalent high 0th control.N=4–10. Figure 2a shows the spectral differences between shear stress from the protective and prone waveforms when a FT is performed [15] . By using FT’s, we can decouple and biologically interrogate the roles of individual harmonics present within the signal. Figure 2: Atheroprone and atheroprotective frequency spectrums regulate NF-κB activity. ( a ) Fourier transform analysis was performed on the protective and prone waveforms. ( b ) The corresponding 0th harmonic (time-average shear stress) from the prone (low 0th) and protective (high 0th) was held constant, while exchanging the higher frequency spectrum from the prone or protective waveforms, or compared with steady flow lacking harmonic content. ( c ) After 24 h of shear stress, NF-κB activity was assessed. Statistics: * P <0.05 for one-way ANOVA, N =8–10, # P <0.05 for Student’s t -test compared with equivalent high 0th control. N =4–10. Full size image As the prone and protective waveforms differ dramatically in both the time-average magnitude of shear stress (0th harmonic) as well as higher harmonics [8] , [11] , we wanted to establish the relative importance of each. To test this, we exposed ECs to (1) the control prone or protective waveforms (both containing naturally occurring frequency content), (2) prone and protective waveforms that exchanged their respective 0th harmonic and (3) a corresponding time-averaged steady shear stress (that is, no frequency content—only the 0th harmonic) ( Fig. 2b ). The data were segmented into low and high 0th harmonic groups from the prone (0.218 dyne cm −2 ) and protective waveforms (14.57 dyne cm −2 ), respectively ( Fig. 2c ). Similar to previous reports, low steady shear stress had greater NF-κB activity compared with the higher magnitude steady flow (grey bars), as did the prone (low 0th, prone spectrum) over the protective (high 0th, protective spectrum) ( Fig. 2c ) [11] , [22] . However, the addition of frequency (prone or protective spectrums compared with steady flow) had a greater effect than simply changing the magnitude in both cases. For the high 0th harmonic conditions, NF-κB activity was insensitive to changes between the prone and protective spectrums. Conversely, at the low 0th harmonic conditions, NF-κB activity was highly dependent on the type of frequency spectrum, indicating that magnitude alone does not account for differences between the two waveforms. This was especially surprising as both waveforms with low 0th harmonics were highly oscillatory (OSI=0.43 and 0.49 for prone and protective spectrum, respectively), indicating that flow reversal alone does not account for signalling differences. Therefore, both the shear stress magnitude and complex frequency content contribute to unique endothelial responses. Fourier ‘mutation’ analysis modulates inflammatory biology We previously reported that the HI, a parameter that describes the relative contribution of the frequency content versus the time-averaged content of haemodynamic waveforms, positively correlated with proatherogenic regions of the human internal carotid artery [15] , [35] ( Fig. 1a ). This suggested that atheroprone regions in vivo are exposed to haemodynamics dominated by the complex frequency content, whereas atheroprotective regions are dominated by the 0th harmonic. We hypothesized that specific frequency components contained in atheroprone and atheroprotective haemodynamics influence the basal inflammatory phenotype in ECs in these regions. To investigate the role of frequency harmonics on the inflammatory endothelial phenotype, we developed a novel method to systematically manipulate individual or sets of harmonics. This new approach has never been explored before, but it is easily within the feasibility and fidelity of our shear stress system. This was done by applying a FT to the control prone and protective waveforms, where in the frequency domain, eight permutations of each waveform were created by exchanging/‘mutating’ harmonics between these two waveforms while maintaining the respective 0th harmonic (that is, time-averaged shear stress) ( Fig. 3a ). Once these mutations were created, an inverse FT was performed to yield a frequency-mutated waveform, where only chosen harmonics are altered and the other components are maintained ( Fig. 3a ). Each of the waveforms was applied to confluent ECs for 24 h and NF-κB activity and downstream inflammatory gene expression were measured. 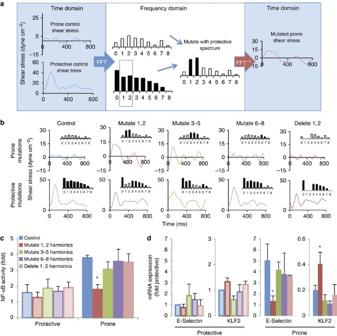Figure 3: Shear stress frequency harmonics contribute to inflammatory phenotype. (a,b) Frequency harmonic content was swapped between control waveforms using Fast Fourier transforms (FFT) to create new ‘mutated’ waveforms for harmonics 1–8. (c,d) The effect of mutating frequency harmonics on NF-κB activity was assessed, along with proinflammatory gene E-Selectin and anti-inflammatory gene, KLF2. Statistics: *P<0.05 for ANOVA (c,d),N=4–7. Figure 3: Shear stress frequency harmonics contribute to inflammatory phenotype. ( a , b ) Frequency harmonic content was swapped between control waveforms using Fast Fourier transforms (FFT) to create new ‘mutated’ waveforms for harmonics 1–8. ( c , d ) The effect of mutating frequency harmonics on NF-κB activity was assessed, along with proinflammatory gene E-Selectin and anti-inflammatory gene, KLF2. Statistics: * P <0.05 for ANOVA ( c , d ), N =4–7. Full size image Frequency mutations in the protective harmonics 1–8 resulted in no change in NF-κB activation relative to its control waveform, and each was significantly lower than the prone control ( Fig. 3c ). No significant changes were seen in either E-Selectin or KLF2 transcription ( Fig. 3d ). However, mutating to the prone waveform by exchanging harmonics 1–2 from the protective waveform significantly blocked NF-κB activation compared with control. The reduction of NF-κB activity correlated with a reduction in proinflammatory E-Selectin gene activation and a significant increase in the atheroprotective transcription factor, KLF2 ( Fig. 3d ). Thus, while no harmonic ‘mutations’ were found to affect the protective waveforms, the 1–2 harmonics were able to block inflammation when altered in the prone condition. The atheroprotective effects observed by exchanging the 1–2 prone harmonics could be due to either (1) the addition of 1st–2nd protective harmonics that attenuate NF-κB activity or (2) the loss of atheroprone frequencies that actively promote NF-κB activity. To test these possibilities, harmonics 1–2 were deleted (that is, set to zero). Figure 3c shows that deleting prone harmonics 1–2 resulted in the same NF-κB activity relative to the control prone waveform. Similarly, no difference was observed when performing the same FT mutation for the protective waveform. Therefore, this novel approach revealed that ‘protective’ harmonics from the protective waveform actively suppress NF-κB activity when present amidst the prone frequency spectrum. As mutating the prone 1–2 harmonics seemed to promote an anti-inflammatory phenotype, a more expansive subset of genes was tested under these conditions. 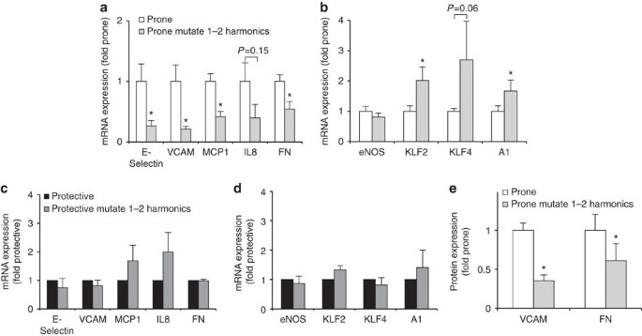Figure 4: Regulation of gene and protein expression by 1–2 harmonic mutation in prone and protective shear stresses. Pro- (a,c) and anti-inflammatory (b,d) genes were assessed after 24 h of control or 1–2 harmonic mutation shear stress. (e) VCAM-1 and FN protein was decreased due to frequency exchanges within the prone waveform. Statistics: *P<0.05 to control paired waveform, Student’st-test (a,b,e) or one-samplet-test (c,d),N=4–7. Figure 4a shows that prone mutations attenuated many atheroprone, NF-κB-dependent genes, including E-Selectin, VCAM-1, MCP-1, IL-8 and FN. VCAM-1 and FN protein levels were also significantly attenuated ( Fig. 4e ). Protective transcription factors, KLF2 and KLF4 and the prosurvival gene A1, were enhanced ( Fig. 4b ). Consistent with the NF-κB profile, downstream genes from the frequency mutations of the protective waveform were unchanged from control ( Fig. 4c ). Overall, mutations in the 1–2 harmonics of the prone waveform promotes an anti-inflammatory phenotype. Figure 4: Regulation of gene and protein expression by 1–2 harmonic mutation in prone and protective shear stresses. Pro- ( a , c ) and anti-inflammatory ( b , d ) genes were assessed after 24 h of control or 1–2 harmonic mutation shear stress. ( e ) VCAM-1 and FN protein was decreased due to frequency exchanges within the prone waveform. Statistics: * P <0.05 to control paired waveform, Student’s t -test ( a , b , e ) or one-sample t -test ( c , d ), N =4–7. Full size image Next, we wanted to determine whether the first and/or second harmonic was responsible for this reduction in NF-κB. To test this, single harmonic mutations were performed on the prone waveform ( Fig. 5a ). Mutating the 1st harmonic alone (M1, Fig. 5c ) lowered the NF-κB activity equivalently to mutating prones 1–2, while swapping just the 2nd resulted in elevated NF-κB activity similar to the prone control ( Fig. 5c ). Therefore, ‘mutations’ where the 1st harmonic from the protective waveform was present in the prone spectrum were sufficient to block NF-κB activity. 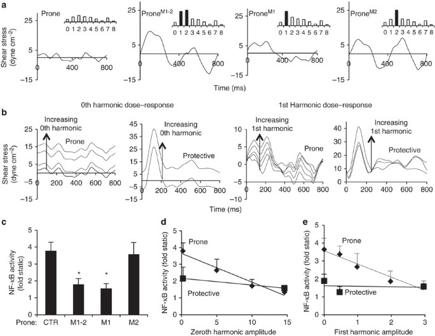Figure 5: Amplitude of the 0th and 1st harmonics regulates NF-κB activity. The effect of shear stress harmonic mutations (a) to the prone 1st (M1), 2nd (M2) or both (M1–2) harmonics on NF-κB activity (c) was compared with the prone control (CTR). Dose increases in the 0th or 1st harmonics in the prone or protective waveforms (b) were selectively generated and applied to ECs for 24 h and NF-κB activity was assessed (d). Statistics: *P<0.05 one-way ANOVA,N=4. Figure 5: Amplitude of the 0th and 1st harmonics regulates NF-κB activity. The effect of shear stress harmonic mutations ( a ) to the prone 1st (M1), 2nd (M2) or both (M1–2) harmonics on NF-κB activity ( c ) was compared with the prone control (CTR). Dose increases in the 0th or 1st harmonics in the prone or protective waveforms ( b ) were selectively generated and applied to ECs for 24 h and NF-κB activity was assessed ( d ). Statistics: * P <0.05 one-way ANOVA, N =4. Full size image To this point we have demonstrated that both the 0th harmonic ( Fig. 2c ) and the 1st harmonic ( Fig. 5c ) individually contribute to a proinflammatory phenotype. To exploit the range of this sensitivity, we tested a ‘dose–response’ to both the 0th and 1st harmonics in the prone and protective waveforms and measured NF-κB activity (see waveforms in Fig. 5b ). Similar to other findings [9] , [11] , we found that increasing the 0th harmonic (that is, time-averaged shear stress) led to a corresponding decrease in NF-κB activity for the prone waveform ( Fig. 5d ). Intriguingly, dose increases in the prone 1st harmonic also reduced NF-κB levels as potently as raising the 0th harmonic, despite each waveform having a low, highly oscillatory shear stress waveform (typically considered proinflammatory) ( Fig. 5e ). NF-κB activity remained low under each protective frequency waveforms, where the dose–responses contained either an elevated 0th and/or 1st harmonic ( Fig. 5d ). Therefore, the atheroprone waveform is more sensitive to changes in the 0th or 1st harmonics, which could individually modulate NF-κB activity. Frequency-based model predicts inflammatory distribution From these studies, two important characteristics have emerged in the activation of NF-κB under complex shear stress waveforms. First, a linear relationship was observed between NF-κB activation and individual changes in the 0th and 1st harmonic within the prone waveform ( Fig. 5 ). Second, there was a nonlinear interaction between these harmonics, as at high 0th harmonics (that is, protective waveform), cells were insensitive to changes in the 1st harmonic ( Fig. 5e ). A linear regression analysis was used to test whether common haemodynamic parameters thought to be indicative of atherogenic shear stress, such as the OSI or HI, significantly correlated with mean experimental NF-κB activity. We found that measures of flow reversal (OSI, number of reversals) and frequency content (HI, 0th and 1st harmonic amplitudes) significantly correlated ( P <0.05) with NF-κB activity, but showed poor predictive capabilities ( R 2 <0.5) ( Supplementary Table S1 , Supplementary Fig. S2 ). Therefore, we developed a regression model that could predict NF-κB activation levels for a given complex, in vivo haemodynamic waveform measured from the circulation using frequency harmonics as the input. To quantitatively assess the role of each of these variables, a least-squares fit was used to fit experimental means from 20 ‘mutated’ and control shear stress waveforms (from Figs. 1 , 2 , 3 , 4 , 5 ) in MATLAB to the following equation that incorporates the above linear and nonlinear characteristics: where A n is the amplitude of the n th harmonic, and constants C n were calculated to minimize error among the data set. By using the above equation, five different models were used to test the relative importance of each term by selectively setting different coefficients ( C n ) to zero and assessing the error and goodness of fit ( Supplementary Table S2 ). We found that the higher-order harmonics were negligible in determining the predictability of the model, and that C 0 – C 3 were necessary for a high R 2 -value and minimal error; thus, the final model ( Fig. 6a or Supplementary Fig. S3 , Model 2) provided the simplest model that accurately predicted NF-κB levels. 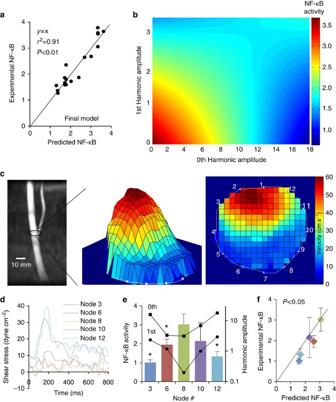Figure 6: A Predictive model for NF-κB activation under physiologic flows. Using 20 different shear stress waveforms, a predictive regression model based on haemodynamic frequency content was generated. (a) The final model of NF-κB activity was able to fit the experimental data. (b) From the final model, a generated colour map shows NF-κB activation as a function of the 0th and 1st harmonic amplitude. (c) Shear stress velocity profiles were measured around the circumference of the carotid sinus via MRI, and the velocity profile was used to calculate wall shear stress around the circumference of the vessel over a cardiac cycle (d). (e) These shear stress waveforms were applied to ECsin vitroand NF-κB activity was assessed (coloured bars) along with the amplitude of the 0th or 1st harmonic (solid lines) at each location. (f) To validate the predictive accuracy of the regression model, harmonic content from these five nodes were used as the input to the regression model to get predicted NF-κB, which was compared with the experimental data. Statistics: *P<0.05 compared with Node 8, one-way ANOVA; ANOVA regression analysis was used to determineP-value for correlation between experimental and predicted NF-κB activity inaand to show that the identity line falls within the 95% confidence interval inf,N=5. Figure 6b shows a colour map of NF-κB activation as a function of the 0th and 1st harmonics from the model. Therefore, an arterial frequency spectrum provides a means of predicting regional NF-κB activation and propensity for disease within the human vasculature. Figure 6: A Predictive model for NF-κB activation under physiologic flows. Using 20 different shear stress waveforms, a predictive regression model based on haemodynamic frequency content was generated. ( a ) The final model of NF-κB activity was able to fit the experimental data. ( b ) From the final model, a generated colour map shows NF-κB activation as a function of the 0th and 1st harmonic amplitude. ( c ) Shear stress velocity profiles were measured around the circumference of the carotid sinus via MRI, and the velocity profile was used to calculate wall shear stress around the circumference of the vessel over a cardiac cycle ( d ). ( e ) These shear stress waveforms were applied to ECs in vitro and NF-κB activity was assessed (coloured bars) along with the amplitude of the 0th or 1st harmonic (solid lines) at each location. ( f ) To validate the predictive accuracy of the regression model, harmonic content from these five nodes were used as the input to the regression model to get predicted NF-κB, which was compared with the experimental data. Statistics: * P <0.05 compared with Node 8, one-way ANOVA; ANOVA regression analysis was used to determine P -value for correlation between experimental and predicted NF-κB activity in a and to show that the identity line falls within the 95% confidence interval in f , N =5. Full size image To test the robustness of this model, we used human haemodynamics previously measured in the carotid sinus of healthy volunteers at equally spaced locations (nodes) around the circumference of the internal carotid artery [15] . Figure 5c shows the three-dimensional cross-sectional peak-velocity profile. The sinus region is located at Node 8 where the shear stress is lowest. Five nodes (nodes 3, 6, 8, 10 and 12) were selected to evaluate the waveforms at those locations in our flow system in vitro ( Fig. 6d ) and NF-κB activity was assessed. Figure 6e shows the NF-κB activity profile of five nodes (bars) around the circumference of the vessel and the 0th and 1st harmonic amplitudes (black lines). It was found that the highest NF-κB activation correlated with the site of the carotid sinus (Node 8), where the 0th and 1st harmonics were at a minimum. Opposite of the sinus (Node 3 and Node 12) had the lowest NF-κB activity and correlated with the highest 0th and 1st harmonic components. Nodes 6 and 8 had similar 0th harmonic amplitudes, but Node 6 had higher 1st harmonic amplitude, which resulted in reduced NF-κB activity. Further, our mathematical model was able to significantly predict the activation of NF-κB within these regions ( Fig. 6f ). These results provide an in vivo -derived example of variations of arterial frequency spectrum that lead to differences in activation of NF-κB, and further supports the hypothesis that differences in regional haemodynamics contribute to proinflammatory phenotype and eccentric development of atherosclerosis. Frequency-dependent regulation of EC inflammation by PECAM-1 Owing to PECAM-1’s established role in mechanotransduction, we tested whether the observed effects on endothelial response to frequency was PECAM-1-dependent. A targeted siRNA approach was used to knockdown PECAM-1 expression (siPECAM: 24±9% PECAM-1 expression relative to siControl) and test its role in frequency sensing under prone flow. Endothelial monolayers were exposed to 24 h of prone control or mutated (1–2 harmonics) haemodynamics. As we found with untransfected cells ( Fig. 3 ), when PECAM-1 was present (siControl), the frequency mutation caused a decrease in NF-κB activity and downstream genes (E-Selectin, MCP-1) and an increase in the anti-inflammatory gene, KLF2 ( Fig. 7a ). However, when PECAM-1 was depleted, this response was reversed; as the frequency mutation caused an increase in NF-κB activity and inflammatory gene expression and a decrease in KLF2 expression ( Fig. 7a ). This result indicates a requirement for PECAM-1 expression in decoding complex haemodynamic frequencies and regulating downstream pathways. 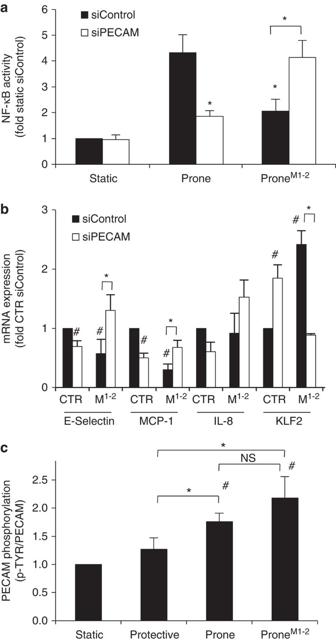Figure 7: PECAM-1 mediates shear stress frequency-dependent NF-κB response. NF-κB activity (a) and gene expression (b) were assessed after 24 h of prone control (CTR) or 1–2 harmonic (M1–2) mutated shear stress for control-treated (siControl) or PECAM-1-depleted (siPECAM-1) ECs. (c) PECAM-1 tyrosine phosphorylation levels were measured relative to static conditions using protective, prone or mutated prone shear stresses. Statistics: *P<0.05 Student’s one-way ANOVA (c), two-way ANOVA (a,b),#P<0.05 one-samplet-test compared with prone control. NS, nonsignificant. Figure 7: PECAM-1 mediates shear stress frequency-dependent NF-κB response. NF-κB activity ( a ) and gene expression ( b ) were assessed after 24 h of prone control (CTR) or 1–2 harmonic (M1–2) mutated shear stress for control-treated (siControl) or PECAM-1-depleted (siPECAM-1) ECs. ( c ) PECAM-1 tyrosine phosphorylation levels were measured relative to static conditions using protective, prone or mutated prone shear stresses. Statistics: * P <0.05 Student’s one-way ANOVA ( c ), two-way ANOVA ( a , b ), # P <0.05 one-sample t -test compared with prone control. NS, nonsignificant. Full size image When PECAM-1 is activated by shear stress, it becomes tyrosine phosphorylated leading to downstream intracellular signalling [36] , [37] . Therefore, we tested whether changes in PECAM-1 phosphorylation occur due to differences in the frequency spectrum and whether this could explain changes in the downstream inflammatory phenotype. Phosphorylated PECAM-1 was detected under all haemodynamic conditions, and phosphorylation was greater under conditions with low 0th harmonics (both prone waveforms) relative to the protective condition with a high 0th harmonic ( Fig. 7c ). Interestingly, ‘mutating’ the prone harmonics did not alter PECAM-1 phosphorylation relative to the control waveform. This indicates that increased PECAM-1 phosphorylation under prone conditions was independent of mutations in the first harmonic, and changes in PECAM-1 phosphorylation alone do not account for its regulation of downstream inflammatory pathways. To our knowledge, this is the first report to show the effect of the frequency spectrum from human haemodynamics on the endothelial response and downstream phenotype. We systematically tested the role of individual frequency harmonics from haemodynamics derived from the human carotid bifurcation on the activation of endothelial NF-κB and pro/anti-inflammatory biomarkers. By mathematically manipulating the haemodynamics’ frequency spectrum and applying them experimentally, it was demonstrated that the 0th and 1st harmonics were capable of ‘tuning’ the endothelial inflammatory response even among the existing frequency spectra. Surprisingly, we found the 1st harmonic to be equally critical as the 0th harmonic in regulating EC phenotype. Higher harmonics likely still contribute to endothelial phenotype, as deleting the 1–2 harmonics, such that harmonics 3–8 dominate, activated NF-κB above steady flow controls. Finally, the frequency spectrum proved to be a superior predictor of vessel wall inflammation, compared with other common haemodynamic parameters (for example, OSI, mean shear stress). Mathematically describing the interactions between frequency harmonics was predictive of regional inflammatory priming between both different arterial regions and eccentrically around the vessel wall. Inflammatory signalling was blocked within all tested waveforms by ‘mutating’ the 0th or 1st harmonic to a higher magnitude, even at lower magnitudes of shear stress. The frequency harmonics affected the expression and deposition of FN, which, we previously demonstrated, sustains a proinflammatory phenotype in atheroprone regions via NF-κB-positive feedback [23] , [24] . Therefore, the downregulation of FN by ‘mutating’ the 1st harmonic may break this cycle and thus contribute to the atheroprotective phenotype. KLF2 and KLF4 are atheroprotective transcription factors that protect the vasculature from atherosclerosis. Both of these genes were upregulated by 0th and 1st harmonics and may comprise important signalling hubs capable of activating a plethora of atheroprotective pathways [3] , [6] , [7] , [38] . Overall, the regional frequency signature may regulate blood vessel health through a number of parallel signalling pathways. The unique combination of frequency harmonics may also have other causal effects on the endothelium and vessel wall. For instance, low 0th harmonics in combination with other frequency harmonics often cause ‘reversing’ shear stress patterns that have been shown to correlate with atherosclerosis. In previous studies, assessing the role of flow reversal has been difficult to decouple, as raising the magnitude of shear stress to remove reversals would also elevate the 0th harmonic (which is protective). We found that reversals alone did not account increased inflammatory signalling in atheroprone regions, as prone controls and 1st harmonic mutations were each highly oscillatory waveforms (OSI >0.40), but with very different NF-κB activity and gene expression ( Figs. 2 , 3 , 4 , 5 , Supplementary Fig. S2 ). Similarly, flow reversal can also increase the residence time (a function of the 0th harmonic and the OSI) [39] of cytokines and other factors in the media; however, control and mutated prone waveforms with similar residence times differed significantly in inflammatory markers, suggesting that mechanotransduction of specific frequency harmonics were more dominant in determining the endothelial inflammatory response, and not flow reversal, per se . These responses are mediated in part by PECAM-1. PECAM-1 sensing of long-term shear stress appears to occur at two different levels: First, PECAM-1 becomes phosphorylated in haemodynamic conditions with low 0th harmonic amplitudes (such as prone). Second, activated PECAM-1 either blocks or stimulates the NF-κB pathway in a frequency-dependent manner. In support of these findings, we previously found scenarios where PECAM-1 had reduced phosphorylation (for example, protective or no flow conditions) and PECAM-1 depletion had no effect on NF-κB activation [22] . When elevated phosphorylation levels were observed (for example, prone control and 1st harmonic mutations), loss of PECAM-1 reversed frequency-dependent effects on the NF-κB pathway. While PECAM-1 seems to be clearly having an important role in shear stress frequency mechanotransduction, these results are complicated by potential residual PECAM-1 signalling due to an incomplete knockdown (reduced by ~75% relative to control) and/or additional mechanosensitive pathways. Thus, PECAM-1 integrates differences in shear stress frequency spectrum and differentially regulates EC phenotype. This is partially supported by Goel et al. [27] , who found that PECAM-1 either promoted or blocked atherosclerotic lesion formation in a site-specific manner in LDLR −/− mice. Perhaps the underlying mechanism is PECAM-1’s long-term integration of differences in the shear stress frequency spectrum in these locations. A body of evidence supports the diverse range of EC phenotypes as dictated by the haemodynamic environment. This study illustrates how site-specific changes in harmonic content controls the cellular inflammatory phenotype. The atheroprotective waveform had both elevated 0th and 1st harmonics that seems to redundantly protect against the development of proinflammatory responses, while the atheroprone is more susceptible due to deficiencies in both. The 0th and 1st harmonics naturally varied eccentrically around the vessel, thus uniquely modulating NF-κB in these regions. Shear stress waveforms may vary from patient-to-patient, but when we tested our findings from circumferential positions of a different subject, we found that the frequency spectrum was still a significant predictor of the inflammatory state ( Fig. 6 ). As MRI blood velocity measurements are non-invasive and accessible, using complex haemodynamics as a biomarker is feasible. Future studies may reveal patients’ propensities to developing disease based on haemodynamic read-outs in addition to biomarkers such as cholesterol, or we may discover unique frequency ‘signatures’ to aid in diagnosis of particular pathologies, such as hypertension, aortic aneurysm or atherosclerotic lesion formation [29] , [40] . Although we focused on inflammation, shear stress frequency spectrums can change under a number of related vascular conditions. For instance, many clinical studies have shown the importance of exercise in the prevention of atherosclerosis. In exercise, changes occur in the fundamental frequency (that is, increased heart rate), as well as, time-averaged shear stress (0th harmonic) due to increased blood flow, among other factors [41] . These changes lead to endothelial activation of protective pathways, such as eNOS [42] . Although an elevated heart rate in exercise is considered atheroprotective, paradoxically, prolonged elevated heart rate has the opposite effect and is associated with increased atherosclerosis [43] . Hypertensive patients have reduced peak and mean wall shear stresses (0th harmonic) within the CCA [44] . This study found that reductions in mean shear stress activate inflammatory pathways, which could contribute to hypertension as a risk factor for atherosclerosis. Vascular biology would greatly benefit by future studies that would include harmonic analysis when measuring alterations in haemodynamics in other disease states, to test whether the findings discovered in this study are universally applicable. The focal nature of endothelial inflammation and atherosclerosis has long been attributed to differences in the local haemodynamic shear stresses, but the precise components of the shear stress signal that contributed to disease were difficult to decouple. Here we show the endothelium’s exquisite sensitivity to small changes in the frequency content of a complex haemodynamic signal and the impact of individual harmonics on the inflammatory state. This knowledge provides a more fundamental understanding and appreciation for the responsiveness of vascular ECs to the haemodynamic environment, and the importance of these environments in inflammation and human disease. Calculation of haemodynamic parameters Shear stress waveforms were previously measured via magnetic resonance imaging (MRI) with an in-plane resolution of 0.18 mm 2 resolution and accurate velocity measuring within 5% from the human circulation in the atheroprone, ICS and the atheroprotective, CCA (ref. 15 ) ( Fig. 1a ). Although this voxel size is relatively large, considering shear stresses vary over length scales considerably smaller—even on the subcellular scale [45] , the spatial resolution of our shear stress profiles is sufficient to capture histological changes in atherosclerosis of the carotid wall (which is routinely visualized by MRI with similar voxel size). Further, these measurements are in agreement with computational fluid dynamics models that have theoretically infinite resolution. The measured magnitude of shear stress is consistent with other MRI and ultrasound-based reports, and MRI has the advantage that it does not rely on assuming a parabolic velocity profiles—an assumption we previously found to not be accurate in the carotid sinus. Thus, we found these waveforms adequate for addressing the hypothesis of this study. Briefly, wall shear stress ( τ wall ) was measured assuming blood was a Newtonian fluid with viscosity ( μ ) of 4 cp around the radius ( r ) of the blood vessel using the following equation: The HI was calculated to assess the relative contributions of harmonics ( A n ) greater than zero compared with the 0th harmonic. As previously, only harmonics 0–3 were significantly different in the carotid artery [15] , these harmonics were considered: Finally, the OSI was calculated: where τ NEG is the shear stress in the direction opposite of the time average from 0 to T (period of the cardiac cycle). This gives a measure of the time spent in reversal, where OSI=0 is unidirectional and OSI=0.5 is purely oscillatory. Frequency mutational analysis As shown in Fig. 3a , using Matlab, a Fast Fourier Transform (FFT) was applied to both shear stress ( τ w ) waveforms in the time domain ( τ w ( t )) ( Fig. 1b ) to yield a representation of shear stress in the frequency domain ( τ w ( ω )) ( Fig. 2a ). The output of the FFT represents relative amplitudes ( A n ) and the phase shift ( ϕ ) for the n th harmonic. Periodic signals, such as the cardiac cycle of shear stress, can be represented as a summation of n sinusoids of pure frequencies (harmonics) in multiples of the fundamental frequency, ω , where: where ω =2π f 0 and ϕ n is the phase angle. The fundamental frequency ( f 0 ) was 1.25 Hz dictated by the resting heartbeat. The coefficients ( A n ) found using the FFT were normalized so that A 0 (the 0th harmonic) is equal to the time average of the waveform. To study the effects of different harmonic content between the prone waveform and the protective waveform, the waveforms underwent a Frequency ‘Mutation’ Analysis (FMA). FMA is defined by the following procedure: (1) the prone or protective waveform was defined in the frequency domain, (2) then individual or multiple harmonics were exchanged (that is, mutated) (prone M , protective M ), deleted (prone D , protective D ) or altered between the waveforms while keeping all other harmonics the same, and finally (3), an inverse FFT was performed to obtain the new ‘mutated’ waveform in the time domain ( Fig. 2a ). This signal in the time domain can be recapitulated using our in vitro flow system. Cell culture Passage two human umbilical vein ECs, isolated as previously described [21] , were plated in M199 growth media (Biowhitaker) supplemented with 10% fetal bovine serum (Hyclone), 5 μg ml −1 EC growth supplement (Biomedical Technologies), 10 μg ml −1 heparin (Sigma), 2 mM L -glutamine (Gibco) and 100 U penicillin/streptomycin (Invitrogen) at 80,000 cells cm −2 on surface-treated plastic coated with 0.1% gelatin and allowed to grow to confluence over 18–24 h. Before flow, cells were washed in DPBS and the medium was exchanged with reduced serum medium (M199 supplemented with 2% fetal bovine serum, 5 μg ml −1 EC growth supplement, 10 μg ml −1 heparin, 2 mM L -glutamine, 100 U penicillin/streptomycin and 4% dextran (w/v) to increase the viscosity) [16] , [17] , [18] , [19] , [20] . In vitro haemodynamic flow model and reagents To investigate the role of shear stress harmonic content on EC phenotype in vitro , a cone and plate flow device imposed shear stress waveforms derived from the human circulation. The flow device provides exchange of fresh medium, as well as a continuously controlled environment to maintain humidity, gas and temperature at 37 °C (ref. 21 ). Immunoprecipitation and western blotting To measure PECAM-1 phosphorylation, cells were collected in ice-cold lysis buffer containing phosphatase and protease inhibitors (Sigma). Samples were immunoprecipitated with 20 μl of anti-PECAM-1 (Santa Cruz) and 50 μl of Dynabead-Protein G according to the manufacturer’s protocol (Invitrogen). After immunoprecipitation, protein was analysed with 4G10 phospho-tyrosine antibody (Upstate) and normalized to total anti-PECAM-1 (Santa Cruz). On completion of the flow experiments, the cells were immediately collected directly into SDS–MAPK sample buffer (Cell Signaling). Western blotting was used to measure relative FN (BD, 1:2,000), VCAM (R&D, 1:500) and PECAM-1 (Santa Cruz, 1:500) protein and normalized to α-tubulin (1:5,000, Sigma-Aldrich) to control for loading. RNA isolation and real-time RT–PCR analysis Total RNA was extracted using PureLink RNA Purification System (Invitrogen) as described by the manufacturer, and reverse transcribed using the iScript cDNA Synthesis Kit (Bio-Rad). Primer sequences for FN, VCAM, E-Selectin, IL-8, MCP-1 and β2-microglobulin have been previously published elsewhere [23] . The expression of mRNA was analysed via real-time reverse transcriptase polymerase chain reaction (RT–PCR) using SYBR master mix (Roche Diagnostics) and an iCycler (Bio-Rad). Viral infection of NF-κB reporter Endothelial cells were infected with five multiplicity of infection adenovirus containing NF-κB-luciferase reporter (Vector Labs) [22] for 16–24 h before the onset of shear stress. At the conclusion of experiments, cells were lysed in cold passive lysis buffer (Promega) and frozen at −80 °C until a luciferase assay was performed. We recognize that there are multiple forms of NF-κB and that promoter binding normally occurs within the cell nucleus. We use ‘NF-κB Activity’ throughout to describe the binding of NF-κB to this reporter construct containing direct repeats of the binding site. siRNA knockdown of PECAM-1 For depleting PECAM-1, ECs were treated with 330 pmol of control (D-001810, Dharmacon) or human PECAM-1 siRNA (L-017029-00, Dharmacon) and 20 μl oligofectamine (Invitrogen) in 3 ml of OptiMEM-I medium for 5 h. Cells were then transferred to fresh medium and incubated for 48 h before flow as previously described [22] . Regression model generation A least-squares fit was used to fit experimental mean data in MATLAB to the following equation: where A n is the amplitude of the n th harmonic and constants C n were calculated to minimize error among the data set. Using the above equation, five different models were used to test the relative importance of each term by selectively setting different coefficients ( C n ) to zero and assessing the error and goodness of fit. Supplementary Table 2 shows the values of the coefficients along with the quality of fit ( R 2 , slope) and error (resnorm=the 2-norm of residual squared calculated by MATLAB). Data analysis and statistics All experimental replicates were normalized to a cell-donor-specific static or flow condition. When means were compared with this control (static, CCA flow or ICS siControls) a one-sample t -test was used to test the null hypothesis that the mean was different from 1. In all other cases, equal variance exists across comparison groups and a one-way analysis of variance (ANOVA) with Tukey’s post-hoc test, two-way ANOVA, and Student’s t -test was performed to evaluate significant differences between means as specified using SigmaStat software with significance being reported at P <0.05. An ANOVA regression was performed to test the correlation of haemodynamic parameters and the mathematical model to experimental NF-κB activity. All values are reported as the mean±s.e. How to cite this article: Feaver, R. E. et al. Human haemodynamic frequency harmonics regulate the inflammatory phenotype of vascular endothelial cells. Nat. Commun. 4:1525 doi: 10.1038/ncomms2530 (2013).